A laboratory study of asymmetric magnetic reconnection in strongly driven plasmas Magnetic reconnection, the annihilation and rearrangement of magnetic fields in a plasma, is a universal phenomenon that frequently occurs when plasmas carrying oppositely directed field lines collide. In most natural circumstances, the collision is asymmetric (the two plasmas having different properties), but laboratory research to date has been limited to symmetric configurations. In addition, the regime of strongly driven magnetic reconnection, where the ram pressure of the plasma dominates the magnetic pressure, as in several astrophysical environments, has also received little experimental attention. Thus, we have designed the experiments to probe reconnection in asymmetric, strongly driven, laser-generated plasmas. Here we show that, in this strongly driven system, the rate of magnetic flux annihilation is dictated by the relative flow velocities of the opposing plasmas and is insensitive to initial asymmetries. In addition, out-of-plane magnetic fields that arise from asymmetries in the three-dimensional plasma geometry have minimal impact on the reconnection rate, due to the strong flows. Magnetic reconnection [1] , [2] is a pervasive phenomenon in the universe. In astrophysics, it is thought to be a key mechanism for energy release in the solar corona and in solar flares, and it is important at the Earth’s dayside magnetopause (see Fig. 1a ). In an earthbound context, it allows for fast reconfiguration of the confining magnetic field and consequent energy loss in magnetized-fusion devices [3] . Reconnection most frequently occurs in these environments, and in fact universally in nature, in configurations where there is an asymmetry in the plasma density, temperature, magnetic field strength, geometry and/or flow across the reconnection layer. In the magnetopause, for example, a strong solar wind drives reconnection across an asymmetric boundary, with differences of a factor of ~0.3 in density and ~7 in magnetic field strength. The plasma thermal β (ratio of thermal to magnetic pressure) is ~0.1 at the high-field, low-density magnetosphere and ~1 at the low-field, high-density magnetosheath and the plasma ram pressure β ram (ratio of ram to magnetic pressure) is ~50 on the solar-wind side, signifying a strongly driven reconnection [4] , [5] , [6] . Despite the prevalence of asymmetry in nature, it is only recently that studies have begun to explore its effects on reconnection, primarily in analytic theory [7] , in numerical simulations of collisional [7] , [8] and collisionless plasmas [9] , [10] , [11] , [12] and in some spacecraft measurements of the Earth’s magnetopause [13] , [14] . 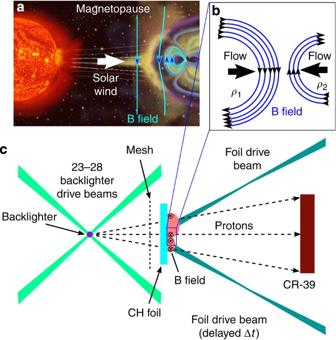Figure 1: Magnetic field configurations and experimental set-up. (a) Magnetic fields at the magnetopause, where the solar wind drives asymmetric reconnection between the interplanetary magnetic field and the Earth’s magnetosphere, bear similarities to (b) magnetic fields and flows in the asymmetric reconnection experiments. (c) In the experiments, the distance between the backlighter capsule and the CH foil was 1 cm, while the distance between the mesh and the foil was 0.2 cm. The distance between the backlighter and the CR-39 proton detector was 27–28 cm, so the magnification wasM=27–28. The relative timing of laser onset of the two foil drive beams was varied from Δt=0 to Δt=0.7 ns. Figure 1: Magnetic field configurations and experimental set-up. ( a ) Magnetic fields at the magnetopause, where the solar wind drives asymmetric reconnection between the interplanetary magnetic field and the Earth’s magnetosphere, bear similarities to ( b ) magnetic fields and flows in the asymmetric reconnection experiments. ( c ) In the experiments, the distance between the backlighter capsule and the CH foil was 1 cm, while the distance between the mesh and the foil was 0.2 cm. The distance between the backlighter and the CR-39 proton detector was 27–28 cm, so the magnification was M =27–28. The relative timing of laser onset of the two foil drive beams was varied from Δ t =0 to Δ t =0.7 ns. Full size image Towards remedying the dearth of experimental investigations of asymmetric magnetic reconnection, here we describe the first concerted, systematic laboratory effort to isolate and study the effects of asymmetry on magnetic reconnection, using strongly driven, colliding, laser-generated plasmas. We demonstrate that, in this strongly driven system, the rate of magnetic flux annihilation in both symmetric and asymmetric experiments is dictated by the relative flow velocities of the colliding plasmas and, therefore, is insensitive to the initial asymmetries in the upstream plasma conditions or in the three-dimensional (3D) geometry of the colliding plasmas. Laser-driven asymmetric magnetic reconnection experiments The experiments were conducted at the OMEGA laser facility [15] . As shown in Fig. 1c , each experiment involved two 500-J beams of 351-nm laser light striking a 5-μm-thick CH foil for 1 ns and focused into 800-μm spots separated by 1.4 mm. The interaction of each laser beam with the foil produced an expanding, hemispherical plasma bubble with an azimuthal 0.5 MG magnetic field concentrated at its perimeter [16] , where the plasma β was around 10. Unlike previous investigations of reconnection in symmetric laser-produced plasma configurations [17] , [18] , [19] , these experiments additionally introduced a delay (Δ t ) between the two beams incident on the foil. This enables the study of the interaction between plasma bubbles that are at different stages in their evolution, with differences in geometry, temperature, density, ram pressure ( , where ρ is the plasma density and V the bulk flow velocity) and magnetic flux. Only the relative timing—no other property—was varied between the two drive lasers, as the magnetic fields and plasma conditions produced by the interaction of a 500-J, 1-ns laser pulse with a 5-μm CH foil have been well characterized by proton radiography and Thomson scattering measurements in previous experiments [20] , [21] . The magnetic Reynolds number R m (a measure of the strength of flow relative to magnetic diffusive processes) is of order 3,000, indicating that the magnetic field was frozen into the flowing plasma, as it is in most astrophysical contexts (where ). Consequently, the magnetic fields were largely advected with the outward radial flow of the plasma bubbles, which expanded into each other and drove their oppositely directed magnetic fields to interact. The resultant magnetic field configuration ( Fig. 1b ) has strong similarities to that of the magnetopause ( Fig. 1a ); a quantitative comparison of plasma conditions and reconnection-relevant parameters for the two contexts is presented in Tables 1 and 2 . Table 1 Plasma parameters for experimental and magnetopause reconnection. 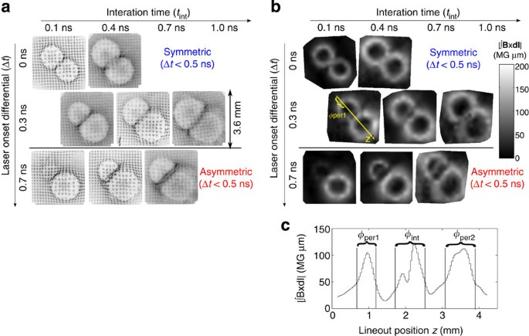Figure 2: Proton radiography data. (a) 15-MeV-proton images and (b) inferred path-integrated magnetic field strength maps at different interaction timestint(since the beginning of bubble interaction) and for differing amounts of bubble asymmetry as parameterized by the laser onset differential Δt(the difference in onset times of the two bubble-generating beams) Each image covers a field of view (at the foil) of 3.6 mm by 3.6 mm. (c) A sample lineout of, is integrated along thezdirection (yellow arrow) to measure the magnetic flux, with limits of integration bracketing each region of interest indicated by the vertical lines. Full size table Table 2 Derived reconnection-relevant parameters. Full size table The magnetic field structures and the rates of magnetic reconnection in the experiments were studied using monoenergetic proton radiography [22] , [23] . The source of the imaging protons (labelled as the ‘Backlighter’ in Fig. 1c ) was fusion reactions of deuterium and helium-3 in an imploding, spherical glass capsule driven by 23 to 28 OMEGA lasers that deliver a total of 11–12 kJ in a 1-ns pulse. The reactions produced an isotropic, ~100-ps burst of monoenergetic 15-MeV protons that were divided into discrete beamlets by a 150-μm-period Ni mesh. The resultant proton radiographs allow measurements of the deflections of individual proton beamlets due to magnetic fields around the laser-produced plasma bubbles, as shown in Fig. 2a , where individual images are organized according to both the duration of time since the plasma bubbles began to interact ( t int ) and the difference in onset time between the two foil drive beams (Δ t ) in the experiment. The absolute time of proton emission from the backlighter was measured using the particle temporal diagnostic [24] . Figure 2: Proton radiography data. ( a ) 15-MeV-proton images and ( b ) inferred path-integrated magnetic field strength maps at different interaction times t int (since the beginning of bubble interaction) and for differing amounts of bubble asymmetry as parameterized by the laser onset differential Δ t (the difference in onset times of the two bubble-generating beams) Each image covers a field of view (at the foil) of 3.6 mm by 3.6 mm. ( c ) A sample lineout of , is integrated along the z direction (yellow arrow) to measure the magnetic flux , with limits of integration bracketing each region of interest indicated by the vertical lines. Full size image Proton radiographs reveal B field dynamics and reconnection The most salient feature in the images of Fig. 2a is the deflection of proton beamlets away from the centre of each bubble due to the azimuthal magnetic field at each bubble’s perimeter. In addition, there are distortions in the beamlet distributions in the image regions corresponding to the interaction of the two bubbles, where there are bubble deformation and reconnection of magnetic fields. In all cases, the proton-path-integrated magnetic field strength can be determined from the magnitude of the beamlet deflections ξ relative to where they would have been in the image plane in the absence of fields: , where m p ( v p ) is the proton mass (velocity), q is the proton charge and A is the foil-detector distance [18] . Resulting maps of path-integrated magnetic field are shown in Fig. 2b . At the later times, most of the field maps show annihilation of magnetic flux and the deformation of magnetic field structures in the reconnection region. The magnetic flux annihilated in the reconnection region was calculated as ΔΦ ann =( Φ per1 + Φ per2 )− Φ int , where Φ per1 and Φ per2 were the fluxes at the perimeters of the individual plasma bubbles and Φ int was the flux measured in the interaction region, where reconnection occurred. The flux in each case was measured as a line-integral of the path-integrated magnetic field strength over the region of interest (see Fig. 2c ) as , where dz is the differential length along the lineout direction, perpendicular to the magnetic fields. The bubble expansion speed V b , as estimated based on the radius of the outer extent of magnetic field structure around an individual bubble, is a relatively constant 450±50 μm ns −1 over the duration of the experiment. This flow velocity is much larger than the nominal Alfvén speed , the speed at which ions can rearrange the magnetic field structure, which is ~100 μm ns −1 at the perimeters of the expanding plasma bubbles just before their collision. Consequently, and in contrast to many previous experiments [25] , magnetic reconnection was strongly driven, with the plasma bubbles driven together faster than the natural velocity at which the magnetic fields can adjust. The measured annihilated flux is compared with the flux advected into the reconnection region based on the constant flow velocity V b in Fig. 3 . This flow-based magnetic flux scales as , where V b is the measured radial expansion velocity; t int is the duration of time since the bubbles began to collide, and is the measured path-integrated magnetic field strength through the perimeter of the smaller bubble. (The larger bubble carries some magnetic fields at a greater height away from the foil than in the smaller bubble, so that some of the magnetic fields of the larger bubble are unopposed by the smaller bubble in the collision process. Thus, the path-integrated field strength that can be annihilated is limited to that contained in the smaller bubble.) In both symmetric and asymmetric cases, the rate of reconnection was nearly equivalent to the flow-based rate, as the flux annihilated Δ Φ ann is . In contrast, this measured rate of flux annihilation is much faster than that based on the nominal Alfvén speed, as Δ Φ ann ~10Δ Φ Alf , where is the amount of flux advected into the reconnection region based on a relative inflow at the Alfvén speed, and the nominal Alfvén speed V A0 ~100 μm ns −1 is based on plasma conditions just before collision in the symmetric experiments (see Table 2 ). This result indicates that the rate of reconnection is much faster than that based on initial, undriven, upstream conditions, demonstrating that flux pileup resulting from the strongly driven collision is likely required to amplify the local magnetic field strength and Alfvén speed to permit reconnection at the flow-based rate. In future experiments, precise, local measurements of the plasma density and magnetic field strength will be obtained to compare local parameters, rather than initial parameters, to the measured rate of magnetic flux annihilation. Such measurements will help evaluate, based on experimentally determined plasma parameters, scaling relations for the reconnection rate under asymmetric conditions, as will be further discussed below in the context of equation (1). Notably, reconnection in the asymmetric experiments was only 20–30% slower than in the symmetric experiments, an essentially insignificant difference. It can, therefore, be concluded that the reconnection rate was governed primarily by the relative velocities of incoming and opposing plasmas, independent of the plasma asymmetry. 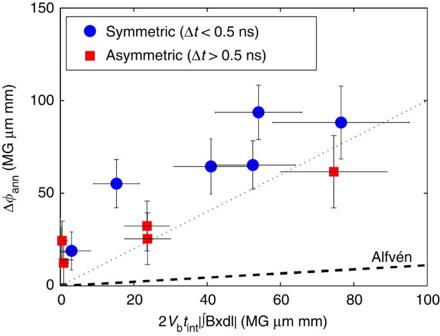Figure 3: Measured annihilated flux. The thin, dotted line denotes the annihilated flux based on the flow velocity, while the thick, dashed line indicates the annihilated flux based on a nominal Alfvénic reconnection rate. Error bars principally denote uncertainty in the boundaries of the magnetic flux regions and the magnitude of proton beamlet deflections. Figure 3: Measured annihilated flux. The thin, dotted line denotes the annihilated flux based on the flow velocity, while the thick, dashed line indicates the annihilated flux based on a nominal Alfvénic reconnection rate . Error bars principally denote uncertainty in the boundaries of the magnetic flux regions and the magnitude of proton beamlet deflections. Full size image Reconnection-relevant plasma parameters Calculation of the plasma parameters in the experiments shows that the magnetic reconnection was strongly driven and that two-fluid effects (decoupled ions and electrons) were important. To estimate the key plasma parameters, we used measurements and simulated quantities from other recent, similar experiments to characterize plasma conditions immediately before collision in a typical, symmetric experiment. These conditions represent the initial conditions in the reconnection region. Though these conditions evolve throughout the experiment, with the density and magnetic field strength likely enhanced early in the collision process, they represent a solid baseline for establishing the regime of these experiments. These parameters are summarized in Tables 1 and 2 . Thomson scattering measurements of local plasma conditions indicated an electron temperature T e =0.7±0.15 keV and an ion temperature of T i =0.3±0.1 keV at the plasma bubble perimeter just before collision in a typical symmetric experiment, at a height of 450 μm away from the foil [21] . The variation in temperature along the collision plane was of order 50% within ±250 μm of this height [21] . The electron density, as predicted by LASNEX radiation-hydrodynamics simulations [26] , [27] of individual laser-produced plasma bubbles, was n e ~5–9 × 10 19 cm −3 within the magnetic field region just before interaction, varying by an additional factor of 2 along the collision plane and increasing by a factor of ~10 towards the centre of the plasma bubbles. On the basis of quasi-neutrality in this fully ionized CH plasma, with an average charge of ‹ Z ›=3.5, the ion density was n i ~1.5–2.5 × 10 19 cm −3 . In addition, the initial magnetic field strength at the perimeter of each bubble, within a ~100 μm-thick ribbon of magnetic fields, was B =0.3–0.5 MG, as predicted by LASNEX and confirmed by experimental data [20] . These numbers imply that the ratio of thermal pressure to magnetic pressure was β ≡( n e kT e + n i kT i )/( B 2 /2 μ 0 )=5–15, while the ratio of ram pressure to magnetic pressure was . It is noted again that the reconnection was strongly driven, by virtue of , or, equivalently, , as previously discussed. The significance of two-fluid reconnection effects in the experiments is assessed by comparing the length scale for electron–ion decoupling to the width of the reconnection region. The ion inertial length, the distance over which electrons and ions decouple in a plasma, was d i ≡c/ ω pi =30–50 μm, where ω pi is the frequency of ion oscillations in a plasma. On the basis of the radiographs, the length L of the boundary layer current sheet was 800±200 μm, while the Lundquist number, the ratio of diffusive to Alfvén timescales, was S ≡ μ 0 LV A0 / η ~450–750, where η is the plasma resistivity. As a result, the current sheet width in the experiments, as predicted by Sweet–Parker reconnection theory [28] , [29] , was and therefore δ SP / d i ~0.9. The ion gyroradius ρ i in the experiment was approximately equal to the ion inertial length of 30–50 μm. On length scales shorter than d i or ρ i , the ions are demagnetized, while the electrons remain tightly bound to the magnetic field lines and electron flow carries magnetic flux into the annihilation region. The conditions in the experiments, with δ SP / d i ≲ 1, were far different from those required for a single-fluid reconnection model, which requires that . All of these parameters evolved with time throughout these highly dynamic experiments, but, on the whole, collisionless or two-fluid effects were important in the reconnection process just as they are in magnetopause reconnection (where electron densities of ~10 cm −3 and magnetic field strengths of ~10 nT imply δ SP / d i ~10 −3 ). Simulations aid and confirm interpretation of measured data To help interpret the physics in these experiments, two-dimensional (2D) numerical simulations were performed. First, the azimuthally symmetric 2D structure and evolution of each individual bubble was simulated with 2D DRACO [30] and LASNEX [31] radiation-hydrodynamics codes. At the point in time when the individual bubbles were about to collide, the conditions in both bubbles (radial profiles of density, temperature, magnetic field strength and flow velocity) on a plane parallel to the foil and 200 μm away from the foil surface were recorded. This height was chosen because it represents the height at which the plasma bubbles initially make contact with each other in the symmetric experiments. The profiles of hydrodynamic quantities—density, temperature and flow velocity—were obtained from DRACO simulations, while magnetic field profiles were qualitatively based on those generated by LASNEX simulations. The DRACO simulations use inverse bremsstrahlung absorption of laser energy and local, flux-limited [32] Spitzer electron heat transport with a flux limiter of f =0.06. Previous laser-foil experiments at a low laser intensity ≲ 2 × 10 14 W cm −2 , relevant to the present experiments, have demonstrated good agreement with DRACO -simulated hydrodynamics [33] . LASNEX simulations use local, flux-limited Spitzer heat flux, with a flux limiter of f =0.1. Though non-local effects were not included in either DRACO or LASNEX , agreement of these models with experimental results under relevant or near-identical experimental conditions [21] suggests that this is not a major limitation. The magnetic field model in LASNEX includes the ∇ T e × ∇ n e source term and convection due to plasma flows and heat-flux (Nernst) effects. These LASNEX simulations did not include Righi–Leduc heat-flux effects, though it has been found that the inclusion of those terms does not significantly modify the hemispherical shape and magnitude of the magnetic field structure. LASNEX simulations identical to those used here have been found to reproduce the path-integrated magnetic field strength in single laser-produced plasma bubbles under conditions identical to the present experiments, producing agreement between proton radiography measurements and synthetic radiographs based on LASNEX -simulated magnetic fields [20] . (To date, DRACO -simulated path-integrated magnetic fields have not been verified in comparison to experimental results as have the LASNEX -simulated path-integrated magnetic fields and so LASNEX -simulated magnetic fields are used.) Electron and ion temperature measurements of individual laser-produced plasma bubbles under identical conditions have also been captured by these LASNEX simulations [21] . Thus, though the out-of-plane field structure has not been directly verified experimentally, these LASNEX simulations are believed to reasonably capture the generation and evolution of magnetic field structure produced in a single laser-foil interaction under these experimental conditions. Analytic fits to separate magnetic field profiles simulated by LASNEX and hydrodynamic profiles simulated by DRACO were then used in concert as initial conditions for further simulation through the bubble interaction phase using the 2D, planar particle-in-cell (PIC) code PSC in a manner previously applied to other experiments involving reconnection in laser-driven plasmas [34] , [35] . Though not perfectly self-consistent, the parameters used to initiate the PIC simulations appropriately capture the strongly driven and high-β regime of the experiments and the physics relevant to the reconnection process. The use of a PIC code, rather than a hydrodynamic code, is necessary during the interaction phase to capture the physics of two-fluid reconnection. The PIC simulations include the effect of collisions through the use of a Monte Carlo collision operator [35] , though collisions do not significantly contribute to the reconnection dynamics. The PIC simulations do not account for continued laser-generation of plasma or of magnetic fields, which artificially stunts the evolution of the small bubble in the asymmetric simulation. These PIC simulations represent a 2D treatment of a fully 3D structure of the hemispherical plasma bubbles and, as such, they do not allow for out-of-plane advection of plasma or fields. This consequently forces a strong collision of magnetic fields. However, the PIC simulations initiated from hydrodynamic codes appropriately capture the physical regime and illuminate key processes dictating the plasma collision and reconnection as they occur in both symmetric and asymmetric experiments. In basic agreement with the data, the PIC simulations show ( Fig. 4 ) the emergence of a reconnection layer in the interaction region, the annihilation of magnetic fields and the deformation of the plasma bubbles due to their hydrodynamic collision. The simulated reconnection rates, expressed in Fig. 4c in terms of the reconnection-related out-of-plane electric field ( E y ), are nearly indistinguishable in the symmetric and asymmetric simulations. This result is consistent with experimental observations. Magnetic field amplification due to flux pileup up to a factor of 4 is observed in the simulations as a consequence of the strongly driven interaction, as in previous modelling studies of related experiments [35] . The simulations show a comparable degree of flux pileup in both symmetric and asymmetric cases, though pileup occurs inversely to the density or ram pressure asymmetry and slightly more weakly overall in the asymmetric simulation. This flux pileup likely explains the fast reconnection rates inferred from the measured magnetic flux data in symmetric and asymmetric experiments. This result indicates, in a manner consistent with prior symmetric simulations [34] and the experimental result discussed above, that the reconnection rate in a strongly driven system is dependent more on the characteristics and strength of the drive mechanism—as determined by the flow velocity—than on ambient plasma conditions and asymmetries. 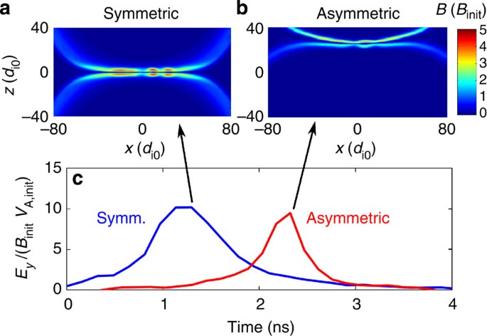Figure 4: 2D PIC simulation results. Simulated magnetic field strength in a plane parallel to the foil at the time of peak reconnection rate for the cases of (a) symmetric and (b) asymmetric interacting plasma bubbles. Spatial units are in terms of a nominal ion skin depthdi0=11 μm and the magnetic field strength is in terms of the peak initial magnetic field strengthBinit=0.5 MG. The simulated reconnection electric fields (c), normalized to initial magnetic field strength and Alfvén speed, are approximately equal in symmetric and asymmetric simulations, consistent with experimental results. The electric field is expressed in terms ofBinitand the nominal Alfvén speedVA,init=31 μm ns−1~1/3VA0in the simulation (based onBinitand the peak simulated densityne,init=6.8 × 1020cm−3), with these scale values used for normalization (seeTable 3). The asymmetric simulation shows a delay in the onset of reconnection, because in this case it takes longer for sufficient pressure to build up on the small-bubble side to push back and drive reconnection. This effect is likely exaggerated in the simulation due to the lack of modelling of the continued laser drive, which in reality increases the pressure on the small-bubble side. Figure 4: 2D PIC simulation results. Simulated magnetic field strength in a plane parallel to the foil at the time of peak reconnection rate for the cases of ( a ) symmetric and ( b ) asymmetric interacting plasma bubbles. Spatial units are in terms of a nominal ion skin depth d i0 =11 μm and the magnetic field strength is in terms of the peak initial magnetic field strength B init =0.5 MG. The simulated reconnection electric fields ( c ), normalized to initial magnetic field strength and Alfvén speed, are approximately equal in symmetric and asymmetric simulations, consistent with experimental results. The electric field is expressed in terms of B init and the nominal Alfvén speed V A,init =31 μm ns −1 ~1/3 V A0 in the simulation (based on B init and the peak simulated density n e,init =6.8 × 10 20 cm −3 ), with these scale values used for normalization (see Table 3 ). The asymmetric simulation shows a delay in the onset of reconnection, because in this case it takes longer for sufficient pressure to build up on the small-bubble side to push back and drive reconnection. This effect is likely exaggerated in the simulation due to the lack of modelling of the continued laser drive, which in reality increases the pressure on the small-bubble side. Full size image The reconnection electric fields are predominantly attributable to the Hall J Hall × B electromotive force and the electron pressure tensor in the current sheet, and they are driven at the periphery of the reconnection region by ion-driven magnetic field advection V i × B . Similar magnitudes of the V i × B term in the symmetric and asymmetric cases arise from the ram pressure around the current sheet, which is approximately equal in the symmetric and asymmetric simulations despite the large asymmetry between the two sides of the current sheet in the asymmetric case. This result suggests that the bulk plasma flows drive electrons to rearrange themselves in a way that produces a strong reconnection electric field and a rapid reconnection, and that this process is largely insensitive to asymmetries. Remarkably, under a wide range of conditions reconnection occurs at the rate implied by the dynamics of the plasma bubble collision, with the local electron behaviour dictated by the strong collision process. The reconnection rate (reconnection electric field) produced in the simulations is also consistent with an analytic theory of asymmetric reconnection [7] based on a ‘hybrid’ Alfvén speed and magnetic field strength—inferred from the local density and magnetic field strength on each side of the current sheet—and the current sheet aspect ratio (opening angle of the reconnection outflow), as where B 1 ( B 2 ) is the magnetic field strength and ρ 1 ( ρ 2 ) is the plasma density on the large (small) bubble side of the current sheet, and δ / L is the current sheet aspect ratio. The hybrid Alfvén speed V A,hybrid is defined [7] as Agreement between the simulated reconnection rates and the predictions of this theory is illustrated based on instantaneous, local conditions around the time of peak reconnection rate. The PIC simulations show that the dynamically evolving asymmetry in the reconnection layer departs significantly from initial asymmetries: primarily, the initial asymmetry is one of plasma density, but as the system evolves and pressure balance is established around the layer the magnetic field asymmetry becomes dominant. At the peak reconnection rate in the symmetric simulation, based on the simulated density of 2.4 × 10 −4 g cm −3 ( n e =7.7 × 10 19 cm −3 for this fully ionized CH plasma), magnetic field strength of 1.7 MG, and current sheet aspect ratio of 0.25, the analytic model predicts E y ~1.4 × 10 7 V m −1 , which compares favourably to the simulated E y ~1.6 × 10 7 V m −1 . Near the peak reconnection rate in the asymmetric simulation, based on simulated densities of 2.0 × 10 −4 g cm −3 ( n e =6.4 × 10 19 cm −3 ; large bubble) and 1.6 × 10 −4 g cm −3 ( n e =5.2 × 10 19 cm −3 ; small bubble), magnetic field strengths of 1.0 and 1.7 MG and an aspect ratio of 0.29, the analytic model predicts E y ~1.0 × 10 7 V m −1 , close to the simulated E y ~0.8 × 10 7 V m −1 at that time. Although agreement with this steady-state model can only be considered suggestive, rather than explanatory, for this strongly driven system, based on the consistency between the equation (1) theory [7] and the PIC simulations, and between the PIC simulations and the measured data, the experimental results provide a rough confirmation of the theory. As was mentioned earlier, a goal of future experiments is to obtain experimental measurements of ρ 1 , ρ 2 , B 1 and B 2 in the reconnection region, to make a direct evaluation of the scaling relation of equation (1) under these strongly driven and dynamic conditions. The picture provided by the experimental results, PIC simulations and equation (1) theory [7] suggests that under such strong external drive, the plasma conditions evolve to permit reconnection at the flow-based rate, regardless of the initial magnetic field, density or ram pressure asymmetry. The concept of ‘driven’ reconnection has been described in previous computational work [36] , including the assertion that the strength of driving flows or the self-consistent out-of-plane electric field can determine the rate of reconnection through modification of local plasma conditions. The results presented here provide strong experimental evidence of this phenomenon in a regime characterized by strong plasma flows and likely flux pileup, with the remarkable observation that magnetic flux is annihilated at nearly exactly the rate dictated by the flow velocities. This property is found to apply generally, for both symmetric and asymmetric conditions across the current sheet. Though recent theoretical work [37] has found that under certain conditions in high-β plasmas, heat flows (rather than Alfvénic flows or, in the case of the present experiments, plasma fluid flows) dictate the reconnection rate, the parameters of these experiments are such that heat-flux effects are small compared to the dominant fluid flow. Heat-flux effects are dominant for a ratio of , where the Hall parameter ω ce τ ei is the product of the electron cyclotron frequecy and the electron–ion collision time. In a computational study [37] at β /( ω ce τ ei )~600–6,000, heat-flux effects were dominant, but for the smaller values of β present in these experiments, β /( ω ce τ ei )~0.1–1 and heat-flux effects are subdominant. The large value of the Hall parameter in these experiments, with ω ce τ ei ~20–40, also indicates that heat conduction perpendicular to the magnetic field is strongly suppressed. This has been confirmed as well in the PIC modelling, which indicates that the flow-related advection of magnetic fields is much greater than the heat-flux (Nernst) magnetic advection. 3D geometry effects have little impact on reconnection rate Though the 3D structure of the plasma bubble collisions is a notable feature of these experiments, in this particular geometry it was found that changes to the magnetic field structures due to a tilt in the reconnection plane and out-of-plane velocity shear have negligible impact on the reconnection rate in this strongly driven case. 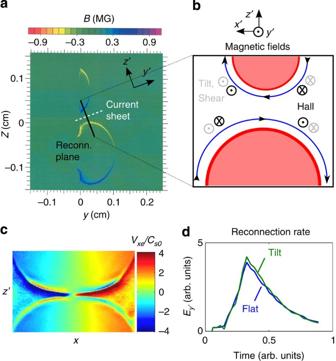Figure 5: Out-of-plane magnetic fields due to 3D effects. (a)LASNEXsimulation of magnetic fields around asymmetric plasma bubbles just before their collision shows (b) how magnetic fields at the reconnection plane are produced, including the quadrupolar Hall magnetic fields (black) and out-of-plane fields due to the tilted reconnection plane and out-of-plane velocity shear across the current sheet (grey). 2D PIC simulations initiated with out-of-plane (‘Tilt’) fields show (c) modified electron flows but (d) a reconnection rate identical to those without external out-of-plane fields (‘Flat’). Figure 5 illustrates two asymmetric plasma bubbles and their magnetic fields just before the collision. Because the bubbles collide in such a way that the reconnection plane ( y ′=0) is not parallel to the foil ( y =0), the azimuthal magnetic fields have a component out of the reconnection plane, forming a bipolar field structure antisymmetric about x ′=0 with a magnitude , where θ is the tilt angle between the foil and the reconnection plane and B 0 ~0.5 MG is the magnitude of the azimuthal magnetic field at the perimeter of each bubble. With θ ~25°, . Figure 5: Out-of-plane magnetic fields due to 3D effects. ( a ) LASNEX simulation of magnetic fields around asymmetric plasma bubbles just before their collision shows ( b ) how magnetic fields at the reconnection plane are produced, including the quadrupolar Hall magnetic fields (black) and out-of-plane fields due to the tilted reconnection plane and out-of-plane velocity shear across the current sheet (grey). 2D PIC simulations initiated with out-of-plane (‘Tilt’) fields show ( c ) modified electron flows but ( d ) a reconnection rate identical to those without external out-of-plane fields (‘Flat’). Full size image In addition, LASNEX simulations indicate that a rapid upward expansion of the small bubble ( V y ,small ~500 μm ns −1 ), in contrast to the weaker upward expansion of the large bubble at the interaction point ( V y ,large ~200 μm ns −1 ), creates a Δ V y ′ ~270 μm ns −1 out-of-plane velocity shear across the current sheet, leading to the generation of additional out-of-plane magnetic fields [38] . For Δ V y ′ ~270 μm ns −1 , B z ′ ~0.4 B 0 , and the velocity shear gradient spread out over ~400 μm, in the same bipolar orientation as that caused by the reconnection plane tilt. Both of these effects are estimated to produce out-of-plane magnetic fields comparable to two-fluid or Hall reconnection out-of-plane magnetic fields (typically 0.1–0.5 B 0 (ref. 35 )) that arise consistently with electron currents, indicating that these additional out-of-plane fields might have been expected to impact the reconnection process. However, based on the data, with reconnection occurring at a similar rate in symmetric and asymmetric experiments, it is inferred that these out-of-plane magnetic fields and their interference with Hall magnetic fields and electron currents have minimal net effect on the reconnection rate. The imposed out-of-plane magnetic fields enhance the electron inflow on the small-bubble side and stymie electron inflow on the large-bubble side due to the J Hall × B tilt force in the - z ′-direction. 2D PIC simulations with additional out-of-plane ‘tilt’ magnetic fields were conducted to assess this effect and have confirmed this result ( Fig. 5c ), demonstrating enhanced electron flow on the upper side of the current sheet, reduced electron flow on the lower side, but no net change in the reconnection rate ( Fig. 5d ). (In contrast, PIC simulations with a quadrupolar out-of-plane magnetic field, opposed to the quadrupolar Hall magnetic fields in each quadrant, show a reconnection rate that is reduced by a factor of ~3.) These ‘tilt’ simulations indicate that typical electron flow speeds related to the Hall current are approximately half of the bulk flow velocity V e ~0.5 V b . It is hypothesized that the minimal impact of the modification of electron flows on the reconnection rate is due to the reconnection process being strongly externally driven, as the small net fractional change in electron velocity Δ V e,net ≲ 0.1 V e from the increase in V e on one side and decrease on the other side is negligible in comparison with the large inflow speeds ( ). Interestingly, these results bear on collisionless guide-field reconnection in strongly driven systems, where small perturbations in the local physics due to out-of-plane fields may be overwhelmed by the strong drive mechanism, in contrast to tenuous, low-β, quasi-steady plasmas [39] . Strongly driven asymmetric magnetic reconnection has been systematically studied in the laboratory using colliding β ~10 laser-produced plasmas. The super-Alfvénic annihilation of magnetic fields is observed to occur at nearly the same, flow-based rate in asymmetric and symmetric experiments. In support of these experiments, 2D PIC simulations indicate that near-equal reconnection electric fields, consistent with local electron physics at the current sheet, is supported and generated by bulk plasma flows into the reconnection region that are nearly equal, on average, in symmetric and asymmetric cases. Out-of-plane magnetic fields, due to the asymmetry in geometry and velocity shear, are predicted to modify electron flow in this two-fluid reconnection event, but are inferred to have minimal impact on the reconnection rate in this experiment. This result is due to the fact that the net change in inflow is small compared to the rapid inflow velocity in this strongly driven system. Strongly driven, two-fluid asymmetric magnetic reconnection such as studied in these experiments occurs in many astrophysics and space physics environments, most notably at the Earth’s dayside magnetopause. The results of these experiments suggest that the rate of reconnection at the magnetopause may be dictated by the strength of the solar wind, which determines the local plasma conditions immediately around the current sheet, and is insensitive to the strongly asymmetric initial plasma conditions far upstream of the reconnection site. Future experiments with different drive conditions may explore a more extensive parameter space of asymmetries in magnetic field strength, density, and drive and directly assess, using locally measured quantities, the predicted reconnection rate scalings. Target and detector information The target foil was 1:1 C:H parylene, with a density of 1.11 g cm −3 . The capsule imploded to produce backlighter protons was a SiO 2 shell with a 420-μm diameter and a 2-μm-thick wall, filled with 18 atm of equimolar deuterium (D)/helium-3 ( 3 He) gas. The Ni mesh was 60 μm thick. 15-MeV backlighter protons are recorded at 100% efficiency as individual tracks deposited in the solid-state nuclear track detector CR-39, filtered by 7.5 μm Ta, ~1,500 μm CR-39 and 200 μm Al. Data processing The CR-39 is etched at 80 °C for 2–3 h in a 6-N solution of NaOH, which reveals the tracks with diameters on the order of ~10 μm. An automated microscope scans and records information about the protons tracks, including their location on the piece of CR-39. Custom software is used to determine track properties and to transform that information into an image of proton fluence incident on the CR-39. The number of proton tracks per area is plotted in Fig. 2a , with the mesh placed between the backlighter source and the experiment producing a grid pattern in proton fluence consisting of an array of individual proton beamlets. A semi-automated Matlab routine identifies the centroid of proton beamlet locations and the orientation and spacing of the unperturbed grid, based primarily on the beamlet points far from the centre that have not been deflected. Connecting beamlets to their original grid point, a map of proton beamlet deflection is constructed. The magnitude of the magnetic field strength integrated along the path of the backlighter proton beamlet is inferred from the magnitude of the beamlet deflection. Modelling parameters The 2D (azimuthally symmetric) DRACO simulations, from which the hydrodynamic profiles of density, temperature and flow velocity were obtained and subsequently fed into the PIC simulations, used a non-uniform Eulerian moving grid, with the highest resolution of 0.25 μm in the direction perpendicular to the foil and 1 μm in the direction parallel to the foil. The time step in the DRACO simulations was around 3 × 10 −14 s (0.03 ps). The LASNEX simulations, from which the approximate magnetic field profiles were obtained and subsequently fed into the PIC simulations, used a 2D, azimuthally symmetric slab geometry composed of arbitrarily shape quadrilaterals. The hydrodynamics was Lagrangian, but in the event of severe grid distortions, the grid was remapped to a more regular shape. These simulations were initiated with a 5-μm thick, 2,000-μm radius foil in a 5,000-μm by 2,000-μm low-density gas background. The gas is used in the simulations for numerical reasons, to give the foil something to expand and rezone into, with a density chosen so that it does not alter the dynamics of the foil. The gas on the laser side had 120 × 210 zones that decreased in size in the direction perpendicular to the foil as the zones got closer to the foil. The back side of the foil had 60 × 210 zones which were also decreased in size closer to the foil. The foil itself had very thin zones in the direction perpendicular to the surface, 0.01 μm on the front and back surfaces, which increased in size up to about 0.3 μm towards the middle of the foil; the radial zone size was 6 μm. In the Lagrangian framework, the zone size evolved with the simulation, so that by 1 ns into the simulation, the smallest zone in the direction perpendicular to the foil was around 1.5 μm wide. The time step was not fixed, and was dynamically determined based on a number of physical processes. Typically, the time step ranged from 0.01 to 1.0 ps during the simulation. The PSC PIC simulations were run as initial value problems, starting with analytic fits to profiles of hydrodynamic quantities such as density, temperature and flow velocity from DRACO simulations and profiles of magnetic field based on LASNEX simulations. The initial electric fields were based on V × B advection and the initial plasma current was fit to self-consistently match the magnetic field profile. The scaling of magnitudes was done to match key dimesionless parameters in the PIC simulation, including: the characteristic electron density ( n e,init ), close to the peak initial density; the characteristic electron temperature ( T e,init ); the peak flow speed ( V init ); the peak magnetic field ( B init ); and length scales associated with profiles of these quantities. The simulations use heavy electrons (electron mass is only 1/100 of the ion mass) and a fairly low speed of light (a factor of 5–10 greater than the characteristic electron thermal speed). These non-physical characteristics force choices to be made in scaling the physical units from DRACO and LASNEX to dimensionless quantities as used in running the PIC simulation. The dimensionless magnetic field magnitude in the PIC simulation is scaled to match the plasma thermal β , while the flow speed magnitude is scaled to match the flow Mach number ( V / C s0 ). The collisionality or resistivity is tuned to match the Lundquist number ( S ), which is equivalent to matching the ratio of the characteristic electron–ion collision rate to electron cyclotron frequency ( ν ei,init / ω ce,init =0.25), where ω ce,init is based on the characteristic magnetic field strength B init . The overall PIC modelling procedure is similar to that described by Fox et al . [35] The global ion skin depth ( d i0 ) is the key unit of length and is based on the characteristic density. The simulation size for the symmetric simulations was 320 × 160 d i0 and for the asymmetric simulations was 320 × 320 d i0 . This difference in size is attributed to a subtle difference in boundary conditions. For both cases, the boundary conditions are double periodic. In the symmetric case, this is equivalent to an infinite chain of plasma bubbles. In the asymmetric case, it is equivalent to an infinite chain of plasma bubble pairs (large and small). The simulation grid was 10,000 × 5,000 for the symmetric simulations and 6,400 × 6,400 for the asymmetric simulations. Approximately 4.5 × 10 9 particles were used, with 400 particles per cell at the characteristic density n e,init . The time steps, expressed in units of the characteristic plasma frequency ω pe,init (based on the characteristic density n e,init ) are d t =0.17/ ω pe,init for the symmetric simulations and n e,init ) are d t =0.27/ ω pe,init for the asymmetric simulations. How to cite this article: Rosenberg, M. J. et al . A laboratory study of asymmetric magnetic reconnection in strongly driven plasmas. Nat. Commun. 6:6190 doi: 10.1038/ncomms7190 (2015). Table 3 Scale parameters for PIC simulations. Full size table